De novo SOX11mutations cause Coffin–Siris syndrome Coffin–Siris syndrome (CSS) is a congenital disorder characterized by growth deficiency, intellectual disability, microcephaly, characteristic facial features and hypoplastic nails of the fifth fingers and/or toes. We previously identified mutations in five genes encoding subunits of the BAF complex, in 55% of CSS patients. Here we perform whole-exome sequencing in additional CSS patients, identifying de novo SOX11 mutations in two patients with a mild CSS phenotype. sox11a / b knockdown in zebrafish causes brain abnormalities, potentially explaining the brain phenotype of CSS. SOX11 is the downstream transcriptional factor of the PAX6–BAF complex, highlighting the importance of the BAF complex and SOX11 transcriptional network in brain development. Coffin–Siris syndrome (CSS; MIM#135900) is a congenital disorder characterized by growth deficiency, intellectual disability, microcephaly, characteristic facial features and hypoplastic nails of the fifth fingers and/or toes ( Supplementary Fig. 1 ). Five subunit genes ( SMARCB1 , SMARCA4 , SMARCE1 , ARID1A and ARID1B ) of the BAF complex (also known in yeast as the SWI/SNF complex [1] ) are mutated in 55–70% of CSS patients [2] , [3] , [4] , [5] , [6] . Mutations in SMARCA2, another BAF complex gene, were reported in the Nicolaides–Baraitser syndrome, which is similar to, but distinct from CSS [7] . Furthermore, de novo PHF6 mutations were found in two CSS patients [6] , although no direct interaction has been reported between the BAF complex and PHF6, which interacts with the nucleosome remodelling and deacetylation complex [6] . As 30–45% of CSS patients were genetically undiagnosed in three large cohort studies [2] , [3] , [4] , [5] , [6] , further genetic investigation is required to fully address the genetic picture of CSS. Here we apply whole-exome sequencing (WES) to 92 CSS patients, and identify two de novo SOX11 mutations in two unrelated patients. sox11 knockdown experiments in zebrafish result in a smaller head and significant mortality, which were partially rescued by human wild-type SOX11 messenger RNA (mRNA), but not by mutant mRNA. WES of CSS patients We identified two de novo SOX11 mutations in two unrelated patients, c.347A>G (p.Tyr116Cys) (in patient 1) and c.178T>C (p.Ser60Pro) (in patient 2) (deposited to LOVD, http://www.LOVD.nl/SOX11 ), among 92 CSS patients (including our previous cohorts [2] , [3] ) analysed by trio-based WES. 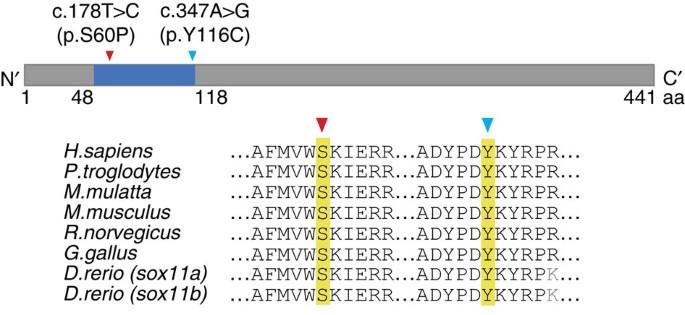Figure 1:SOX11mutations and functional characterization. SOX11mutations in CSS patients. Two missense mutations in the HMG domain (blue box) occur at evolutionarily conserved amino acids. In the two patients, >10 reads covered 94–92% of coding sequences and only SOX11 mutations remained as candidate variants in both of them based on the de novo model with scores of damaging or disease causing by SIFT, PolyPhen2 and Mutation Taster ( Supplementary Table 1 ). The two heterozygous mutations localize to the high-mobility group (HMG) domain. Neither mutation was registered in the databases examined (1,000 Genomes, Exome Sequencing project (ESP) 6500, and in-house databases containing 575 control exomes) ( Supplementary Table 1 ). We identified a further 22 SOX11 variants within these three databases, but all of them reside outside the HMG domain and, based on prediction programs, are less likely to be pathogenic ( Supplementary Table 1 ; Supplementary Fig. 2 ). The amino acids altered in SOX11 are evolutionarily conserved from zebrafish to human ( Fig. 1 ). The mutations do not alter nuclear localization of SOX11 protein ( Supplementary Fig. 3 ). De novo mutations were confirmed in the two families by Sanger sequencing along with biological parentage. No mutations in any of the other BAF complex genes, PHF6 , or other potential candidate genes were found in the two families. Therefore, the two mutations identified are highly likely to be pathogenic. Moreover, SOX11 was sequenced by WES ( n =23) or Sanger method ( n =67) in a further 90 CSS patients, with no mutations found. Fifty-four patients had a mutation in one of the five BAF complex subunit genes (58.7%) ( SMARCA4, SMARCB1, SMARCE1, ARID1A and ARID1B mutations found in 9, 8, 1, 5 and 31 patients, respectively). Figure 1: SOX11 mutations and functional characterization. SOX11 mutations in CSS patients. Two missense mutations in the HMG domain (blue box) occur at evolutionarily conserved amino acids. Full size image Clinical features of patients with SOX11 mutations The two patients showed dysmorphic facial features, microcephaly, growth deficiency, hypoplastic fifth toe nails and mild intellectual disability [8] ( Supplementary Fig. 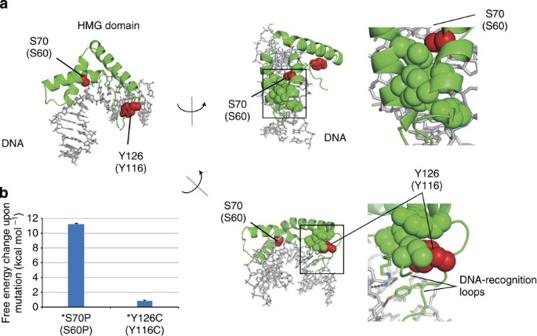Figure 2: Structural effects of SOX11 mutations. (a) Crystal structure of the mouse Sox4 HMG domain bound to DNA. Helices and loops are shown as green ribbons and threads, respectively. DNA is shown as grey sticks. Amino-acid residues at mutation sites are shown coloured red in the space-filling model. In the middle and right images, some of the amino-acid residues involved in the hydrophobic core surrounding mutation points are shown coloured green in the space-filling model. Amino-acid numbering is indicated for mouse Sox4 with that for human SOX11 in parentheses. Hydrogen bonds are shown as black dotted lines. Molecular structures were drawn using PyMOL (http://www.pymol.org). (b) Free energy changes on the indicated mutations calculated by FoldX software. 1 ; Supplementary Table 2 ). The observed clinical features in both patients are classified to a mild end of CSS as patient 1 spoke early for CSS and patient 2 has relatively high intelligence quotient. Although the two patients do not look similar in facial appearance (patient 1 has midface hypoplasia, while patient 2 does not; in addition there is an ethnic difference, as patients were either Japanese or Indian), they do share features in common, namely, hypertrichosis, arched eyebrows, low-set ears, auricular back-rotationand full cheeks ( Supplementary Fig. 1 ). Patient 1 (Japanese) was born at 38 weeks of gestation following an uneventful pregnancy. Her birth weight was 2,340 g (−1.9 s.d. ), length 45 cm (−2.2 s.d.) and occipitofrontal circumference (OFC) 30.5 cm (−1.8 s.d.). She was hypotonic, had feeding difficulties (especially during the neonatal period) and delayed development. She was able to support her head at 5 months of age, sit at 11 months and walk independently at 1 year 11 months. She started to speak meaningful words at 1 year 7 months. At 3 years, her developmental quotient was estimated using the Kyoto scale of psychological development to be 57. Abdominal echography showed her left kidney was slightly small in size. She has distinctive facial features characterized by midface hypoplasia, short palpebral fissures, hypertelorism, upturned palpebral fissures, long eyelashes, a low nasal root, shortened nose with upturned nostrils, short philtrum, open mouth, full lips and low-set ears. Hypoplastic distal phalanges with nail hypoplasia (especially of the fifth digits) were also noted. Additional findings included hypertrichosis and long eyelashes with abundant hair on the scalp. At 4 years 8 months, she was short with a height of 92.1 cm (−2.9 s.d.) and evaluated for possible growth hormone deficiency with stimulation tests, which showed normal results. At 10 years, she measured 119 cm (−2.8 s.d. ), weighed 20.1 kg (−1.8 s.d.) and had an OFC of 47.3 cm (−3.3 s.d.). She attends a special education class for poor performance, but can walk to school by herself (takes approximately half an hour) and is able to communicate verbally, to some extent, with her classmates. Clinical features are summarized in Supplementary Table 2 . Patient 2 (Indian) is a 16-year-old female, and was referred to the genetics outpatient department for evaluation of short stature. She was born at term following a normal pregnancy, but with low birth weight (1.75 kg, −4s.d.). Developmental milestones were attained normally, but her parents always felt that she lagged behind other children. She was a slow learner with poor scholastic performance and an intelligence quotient of 70–80. She attended a normal class, but struggled to pass class examinations every year. She has a proportionately short stature but not a coarse face. Her chin was small and supraorbital ridges hypoplastic with no ptosis. Her nose was long and alae nasi hypoplastic with overhanging columella. Her hair was thick and rough with some thinning on her scalp. She had increased hair on her back. Her fourth and fifth toes were short and all her finger nails were hypoplastic with thin and tapered fingers. Her fourth and fifth toes on both feet, and also the third toe on her right foot, were markedly hypoplastic. Clinodactyly was noted on the third, fourth and fifth toes on her right foot, and the third and fourth toes on her left foot. A skeletal survey did not show any radiographic bone abnormalities. Her bone age was 13–14 years and follicle-stimulating hormone was 1.57 IU l −1 (normal range: <5 IU l −1 ). Ultrasonographic examination at 16 years (before menarche), showed a hypoplastic uterus and malrotation of both kidneys. No secondary sexual characteristics were recognized until she had menarche at 17 years. Now at age of 17 years, she is still short with a height of 141 cm (−5 s.d. ), weigh 31.3 kg (−3 s.d.) and OFC 50.5 cm (−4.5 s.d.). Clinical features are summarized in Supplementary Table 2 . Structural effects of SOX11 mutations To determine the impact of the disease-causing mutations on human SOX11 structure and function, we mapped the mutation positions onto the crystal structure of mouse Sox4 [9] , that is analogous to human SOX11, and calculated free energy changes on the mutations using FoldX software [10] , [11] . The mutations lie in the highly conserved HMG domain, responsible for sequence-specific DNA binding ( Fig. 2a ) [9] . Ser60 is located in a helix of the HMG domain ( Fig. 2a ), therefore the S60P mutation may affect overall folding of the HMG domain and impair DNA binding of SOX11. FoldX calculations supported this prediction and the free energy change on the mutation was high enough to destabilize protein folding (>10 kcal mol −1 ) ( Fig. 2b ) [12] . Conversely, Tyr116 forms a hydrophobic core with the side chains of DNA-recognition loops ( Fig. 2a ). The Y116C mutation has low free energy change (<1 kcal mol −1 ) ( Fig. 2b ), and is unlikely to significantly affect folding of the HMG domain, but instead may alter conformation of the DNA-recognition loop, which is important for DNA binding. Figure 2: Structural effects of SOX11 mutations. ( a ) Crystal structure of the mouse Sox4 HMG domain bound to DNA. Helices and loops are shown as green ribbons and threads, respectively. DNA is shown as grey sticks. Amino-acid residues at mutation sites are shown coloured red in the space-filling model. In the middle and right images, some of the amino-acid residues involved in the hydrophobic core surrounding mutation points are shown coloured green in the space-filling model. Amino-acid numbering is indicated for mouse Sox4 with that for human SOX11 in parentheses. Hydrogen bonds are shown as black dotted lines. Molecular structures were drawn using PyMOL ( http://www.pymol.org ). ( b ) Free energy changes on the indicated mutations calculated by FoldX software. Full size image SOX11 mutations affect downstream transcription Both mutations are located within the HMG domain, which is required for SOX11 transcriptional regulation of GDF5 (ref. 13 ). Luciferase assays using the GDF5 promoter in HeLa and ATDC5 cells, showed both mutant proteins had decreased transcriptional activities compared with wild type (WT) ( Fig. 3 ). 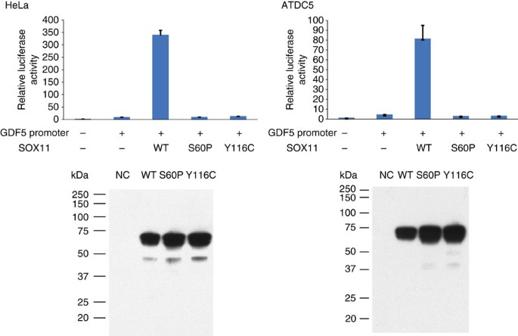Figure 3:SOX11mutations affectingGDF5promoter activity. Luciferase reporter assays measured transcriptional activity of theGDF5promoter (−448/+319) (UCSC genome browser hg19: chr20: 34025709-34026457) in HeLa (left) and ATDC5 (right) cells. HeLa or ATDC5 cells were co-transfected with WT or mutant (S60P and Y116C) SOX11 expression vector and reporter constructs containing either GDF5 promoter or empty vector (pGL3-basic). Relative luciferase activities compared with empty vector are presented as mean±s.d. for two independent experiments, with each experiment performed in triplicate (upper). Immunoblot analysis of transfected HeLa and ATDC5 cell extracts showing wild-type (WT) or mutant (S60P and Y116C) SOX11 proteins (lower). Compared with WT, both SOX11 mutants reducedGDF5transcriptional activities in HeLa and ATDC5 cells. Figure 3: SOX11 mutations affecting GDF5 promoter activity. Luciferase reporter assays measured transcriptional activity of the GDF5 promoter (−448/+319) (UCSC genome browser hg19: chr20: 34025709-34026457) in HeLa (left) and ATDC5 (right) cells. HeLa or ATDC5 cells were co-transfected with WT or mutant (S60P and Y116C) SOX11 expression vector and reporter constructs containing either GDF5 promoter or empty vector (pGL3-basic). Relative luciferase activities compared with empty vector are presented as mean±s.d. for two independent experiments, with each experiment performed in triplicate (upper). Immunoblot analysis of transfected HeLa and ATDC5 cell extracts showing wild-type (WT) or mutant (S60P and Y116C) SOX11 proteins (lower). Compared with WT, both SOX11 mutants reduced GDF5 transcriptional activities in HeLa and ATDC5 cells. Full size image SOX11 expression SOX11 transcription levels were examined using multiple human complementary DNA (cDNA) panels. SOX11 was exclusively expressed in brain (foetus and adult) and heart (adult) tissues, supporting a role for SOX11 mutations in the brain features of CSS observed in the two patients ( Supplementary Fig. 4 ; Supplementary Table 2 ). In mice, targeted Sox11 disruption with a β-galactosidase marker gene results in 23% birth weight reduction and lethality after the first postnatal week in homozygotes, due to hypoplastic lungs and ventricular septation defects. In addition, skeletal malformations (including phalanges) and abdominal defects are observed [14] . Physical and functional abnormalities in heterozygotes have not been described. However, in heterozygous mice, β-galactosidase expression revealed early ubiquitous expression throughout the embryo with upregulation in the central nervous system (CNS) and limb buds [14] . sox11 knockdown experiments in zebrafish We further investigated sox11 function in zebrafish. The zebrafish genome contains two orthologs of human SOX11 , sox11a and sox11b , which are expressed in all cells until gastrulation and later become restricted to the developing CNS [15] , [16] . We knocked down zebrafish sox11a and sox11b (both single-exon genes) using translation-blocking morpholino oligonucleotides (MOs) ( sox11a -MO, sox11b -MO and sox11a/b -MO), as previously described [17] ( Supplementary Fig. 5a ). Off-target effects of morpholino injections were excluded by repeated experiments, co-injecting with tp53 MO or injecting into tp53 zdf1/zdf1 mutant fish [18] , [19] . sox11a - and sox11b -MO knockdown caused similar phenotypes, including smaller heads and body curvature ( Supplementary Fig. 5b ). Low-dose sox11a - (1.6 ng), sox11b - (1.6 ng) and sox11a/b - (1.6 ng) MO-injected embryos resulted in significant mortality ( sox11a -MO, ~49.3%; sox11b -MO, ~19.3%; sox11a/b -MO, ~53.0%), compared with control-MO embryos (~7.3%) ( Fig. 4a ). Co-injection of WT human SOX11 mRNA (h SOX11 -WT mRNA) with sox11a/b -MO improved morphant survival at 48 h post fertilization (hpf) (25.5% lethality versus 49.3% lethality with sox11a/b -MO alone) ( P <0.01) ( Fig. 4a ; Supplementary Fig. 5c ). The affected phenotype of sox11a/b double morphants was partially rescued by h SOX11 -WT mRNA overexpression (4.5% normal for sox11a/b -MO alone versus 36.5% for co-injection with h SOX11 -WT mRNA and sox11a/b -MO, P <0.01) ( Fig. 4a ). In contrast, co-injection of either mutant h SOX11 mRNA (h SOX11 -S60P and -Y116C mRNA) with sox11a/b -MO showed no significant rescue effects on lethal and affected phenotypes ( Fig. 4a ). There were significantly more normal phenotypes following h SOX11 -WT mRNA and sox11a/b -MO co-injection, than with h SOX11 -mutant mRNA co-injections ( P <0.05). Head sizes in randomly selected embryos ( n ≥10) of sox11a and sox11a/b morphants at 48 hpf were significantly decreased ( P <0.05 in both), but not significantly changed in sox11b morphant. Overexpression of h SOX11 -WT mRNA restores sox11a/b double-morphant head size (in randomly selected embryos, n ≥10), suggesting specific sox11 suppression by morpholino injection ( Fig. 4b ). Although the head size of h SOX11 -mutant mRNA and sox11a/b -MO-injected embryos was slightly decreased, no significant difference was recognized between overexpression of h SOX11 -WT or h SOX11 -mutant mRNA and sox11a/b -MO co-injection ( Fig. 4b ).Staining with acridine orange and terminal deoxynucleotidyl TdT-mediated dUTP nick end labelling (TUNEL), found significant apoptotic increases exclusively in microcephalic embryos ( Fig. 4c ; Supplementary Fig. 6 ). Brain cell death was prevented by co-injection with h SOX11 -WT mRNA, but not by mutant h SOX11 mRNAs ( Fig. 4c ). We also used HuC/D (a marker for early postmitotic and mature neurons) and acetylated tubulin (an axonal marker) immunostaining at 48 hpf to analyse neuronal cells in more detail ( Supplementary Fig. 7 ). Decreased HuC/D-positive neurons, especially in the telencephalon and diencephalon, were observed in sox11 morphants ( Supplementary Fig. 7a ). The phenotype in sox11a/b -MO-injected embryos was efficiently rescued by h SOX11 -WT mRNA ( Supplementary Fig. 7a ). Reduction of HuC/D-positive neurons was unaltered by mutant h SOX11 mRNA overexpression and sox11a/b -MO injection ( Supplementary Fig. 7a ). Anti-acetylated tubulin staining also showed severely reduced axonal numbers in the forebrain, midbrain and hindbrain of sox11 morphants, compared with control-MO-injected embryos ( Supplementary Fig. 7b ). sox11a/b morphants showed phenotypic rescue when co-injected with h SOX11 -WT mRNA, compared with mutant h SOX11 mRNAs ( Supplementary Fig. 7b ). 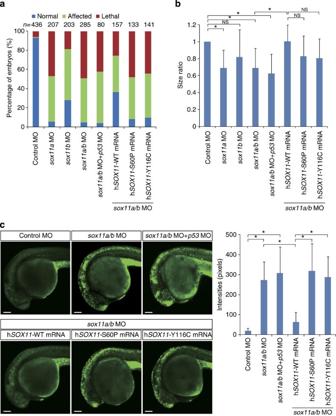Figure 4:sox11a/bknockdown experiments in zebrafish. (a) Embryos were injected withsox11-MO alone or withsox11- andtp53-MO or withsox11-MO andin vitrotranscribed humanSOX11(hSOX11) mRNA (WT, wild type; S60P, p.Ser60Pro; Y116C, p.Tyr116Cys). Injected embryos were categorized as normal, affected and lethal at 48 hpf. The lethal and affected phenotype insox11a/b-MO-injected embryos was partially rescued by WT hSOX11mRNA overexpression. All experiments were performed more than twice and evaluated statistically with a Student’st-test. (b) Head size ratios of embryos with control-,sox11a-,sox11b- orsox11a/b-MO alone, or withsox11a/b- andtp53-MO orsox11a/b-MO and hSOX11mRNA (WT or mutant) at 48 hpf (n≥10) (average of control-MO as 1). Dorsal views of midbrain width were measured. Data are represented as mean±s.d. *P<0.05 by Student’st-test. NS, not significant. (c) Brain cell death in MO-injected embryos at 30 hpf using acridine orange staining (lateral view).sox11morphants show increased cell death in the CNS. Scale bar, 100 μm. Quantification of acridine orange intensities in morphants are shown graphically (right,n≥10). Data are represented as mean±s.d. *P<0.001 by Student’st-test. Figure 4: sox11a / b knockdown experiments in zebrafish. ( a ) Embryos were injected with sox11 -MO alone or with sox11 - and tp53 -MO or with sox11 -MO and in vitro transcribed human SOX11 (h SOX11 ) mRNA (WT, wild type; S60P, p.Ser60Pro; Y116C, p.Tyr116Cys). Injected embryos were categorized as normal, affected and lethal at 48 hpf. The lethal and affected phenotype in sox11a/b -MO-injected embryos was partially rescued by WT h SOX11 mRNA overexpression. All experiments were performed more than twice and evaluated statistically with a Student’s t -test. ( b ) Head size ratios of embryos with control-, sox11a -, sox11b - or sox11a/b -MO alone, or with sox11a/b - and tp53 -MO or sox11a/b -MO and h SOX11 mRNA (WT or mutant) at 48 hpf ( n ≥10) (average of control-MO as 1). Dorsal views of midbrain width were measured. Data are represented as mean±s.d. * P <0.05 by Student’s t -test. NS, not significant. ( c ) Brain cell death in MO-injected embryos at 30 hpf using acridine orange staining (lateral view). sox11 morphants show increased cell death in the CNS. Scale bar, 100 μm. Quantification of acridine orange intensities in morphants are shown graphically (right, n ≥10). Data are represented as mean±s.d. * P <0.001 by Student’s t -test. Full size image We have identified SOX11 mutations in CSS. This is the first report of human mutations in SOXC ( SOX4 , SOX11 and SOX12 ) [20] . SOX11 / sox11 is required for neurogenesis, and loss of function in early embryos is sufficient to impair normal CNS development. Haploinsufficiency of other SOX genes ( SOX2 , SOX9 and SOX10 ) is known to cause human diseases [21] , [22] , [23] . It is interesting that mutations of SOX11 and other BAF subunit genes are mutually exclusive in CSS. Sox11 was recently shown to form a transcriptional cross-regulatory network downstream of the Pax6–BAF complex. The network drives neurogenesis and converts postnatal glia into neurons [24] . Brg1 (Smarca4) binds to the Sox11 promoter, and interaction with Pax6 is sufficient to induce Sox11 expression in neurosphere-derived cells in a Brg1-dependent manner [24] . Therefore, the Pax6–BAF complex activates a cross-regulatory transcriptional network, maintaining high expression of genes involved in neuronal differentiation and execution of cell lineage decisions [24] . SOX11 mutations appear to be a rare cause of CSS as only 2 out of 92 patients (2.2%) showed SOX11 abnormality and to be limited to the mild end of CSS phenotype. Abnormality of the upstream BAF complex tends to show a more severe phenotype compared with that of a downstream SOX11 mutation, which may indicate rather specific effects of SOX11 mutations on the CSS phenotype. In conclusion, mutations in both BAF complex genes and SOX11 result in the same phenotype (CSS), providing strong support for the BAF complex and SOX11 function in a common pathway, and play an important role in human brain development. Subjects and clinical data Patients were seen by their attending clinical geneticists. DNA samples were isolated from peripheral blood leukocytes using standard methods. Informed consent was obtained from the parents of the patients for experimental protocols and displaying participants’ facial appearances in publications. This study was approved by the institutional review board of Yokohama City University School of Medicine. A total of 92 patients were analysed, including 71 patients from a previous cohort and 21 new patients. WES Trio-based WES was performed in two families. Briefly, 3 μg of genomic DNA was sheared using the Covaris 2S system (Covaris, Woburn, MA) and partitioned using SureSelect Human All Exon V4 or V4+UTRs (Agilent Technology, Santa Clara, CA), according to the manufacturer’s instructions. Exon-enriched DNA libraries were sequenced using HiSeq2000 (Illumina, San Diego, CA) with 101-bp paired-end reads and 7-bp index reads. Four samples (2.5 pM each, with different indexes) were run in one lane. Image analysis and base calling were performed using HiSeq Control Software/Real-Time Analysis and CASAVA1.8.2 (Illumina). Mapping to human genome hg19 was performed using Novoalign ( http://www.novocraft.com/main/page.php?s=novoalign ). Aligned reads were processed by Picard ( http://picard.sourceforge.net ) to remove PCR duplicates. Variants were called using the Genome Analysis Toolkit 1.5–21 (GATK v3) with best practice variant detection ( http://gatkforums.broadinstitute.org/discussion/15/best-practice-variant-detection-with-the-gatk-v1-x-retired ), and annotated by Annovar (23 February 2012) ( http://www.openbioinformatics.org/annovar/ ). Common variants registered in dbSNP137 (MAF≥0.01) ( http://genome.ucsc.edu/cgi-bin/hgTrackUi?hgsid=281702941&c=chr1&g=snp137Flagged ) were removed. Prioritization of variants From all the variants within exons and ±2 bp of intronic regions from exon–intron boundaries, those registered in either dbSNP137, 1,000 Genomes ( http://www.1000genomes.org/ ), ESP 6500 ( http://evs.gs.washington.edu/EVS/ ) or our in-house (exome data from 408 individuals) databases, and those located within segmental duplications, were removed and we focused on heterozygous non-synonymous and splice site variants, which were subsequently confirmed by Sanger sequencing. SOX11 mutations in LOVD, http://www.LOVD.nl/SOX11 . Structural modelling and free energy calculations The crystal structure of the mouse Sox4 HMG domain bound to DNA (Protein Data Bank code 3U2B) was selected by SWISS-MODEL server 5 (ref. 25 ) as the structure most resembling human SOX11. To examine the missense mutations, mutational free energy changes were calculated using FoldX software (version 3.0) [10] , [11] . Calculations were repeated three times, and resultant data presented as average values with s.d. SOX11 expression analysis in human tissues TaqMan quantitative real-time PCR was performed using cDNAs from adult (Human MTC Panel I, #636742, Clontech Laboratories, Mountain View, CA) and foetus (Human Fetal MTC Panel, #636747, Clontech Laboratories). Pre-designed TaqMan probes for human SOX11 (Hs00167060_m1, Life Technologies Co., Carlsbad, CA) and human beta-actin (ACTB, 4326315E, Life Technologies Co.) were used. PCR was performed on a Rotor-Gene Q (QIAGEN, Valencia, CA) and expression levels normalized to ACTB , an internal standard gene, according to the 2 −ΔΔCt method. Kidney expression was used as the standard (1 × ). Expression vectors The SOX11 open-reading frame clone was purchased from Promega (Tokyo, Japan) and SOX11 mutants (c.178T>C; p.Ser60Pro and c.347A>G; p.Tyr116Cys) generated by site-directed mutagenesis with the KOD-Plus-Mutagenesis Kit (TOYOBO, Osaka, Japan). WT and mutant SOX11 cDNAs were PCR amplified and cloned into the pEF6/V5-His B mammalian expression vector (Life Technologies) using the In-Fusion PCR Cloning Kit (Clontech Laboratories), and also into the p3xFLAG-CMV-14 mammalian expression vector (Sigma, St Louis, MO). The GDF5 promoter 5′-flanking sequence (−448/+319) was PCR amplified and cloned into the pGL3-basic vector (Promega). All constructs were verified by Sanger sequencing. Human SOX11 cDNA can be obtained from GenBank/EMBL/DDBJ nucleotide core database under the accession code AB028641.1 . Immunostaining Mouse neuroblastoma 2A (Neuro-2A) cells were cultured in Dulbecco’s modified Eagle’s medium (DMEM)–high glucose GlutaMAX supplemented with 10% fetal bovine serum (FBS) and penicillin-streptomycin (Life Technologies Co.). Neuro-2A cells were plated into 24-well plates, 24 h before transfection. Each expression construct (200 ng) was transfected into Neuro-2A cells using X-tremeGENE 9 DNA Transfection Reagent (Roche Diagnostics, Indianapolis, IN). Twenty-four hours after transfection, cells were fixed in 4% paraformaldehyde (PFA)/phosphate-buffered saline (PBS) for 15 min at room temperature, and permeabilized in 0.1% Triton X-100/PBS for 5 min at room temperature. C-terminal V5-6xHis-tagged SOX11 proteins were detected using a mouse anti-V5 primary antibody (1:200; Life Technologies Co.) and an Alexa Fluor 546 Goat Anti-Mouse IgG secondary antibody (1:1,000; Life Technologies Co.). Smears were mounted in Vectashield mounting medium with DAPI (Vector Lab., Burlingame, CA). Confocal images were acquired using a Fluoview FV1000-D microscope (Olympus, Tokyo, Japan). Luciferase assay HeLa cells were cultured in DMEM-high glucose supplemented with penicillin (50 units ml −1 ), streptomycin (50 μg ml −1 ) and 10% FBS. ATDC5 cells were cultured in DMEM/Ham’s F-12 (1:1) supplemented with the above antibiotics and 5% FBS. Cells were plated in 24-well plates, 24 h before transfection, and transfections performed using TransIT-LT1 (Takara, Ohtsu, Japan) with pGL3 reporter (500 ng per well), effector (250 ng per well) and pRL-SV40 internal control (6 ng per well) vectors. Twenty-four hours after transfection, cells were harvested and luciferase activities measured using the PicaGene Dual SeaPansy Luminescence Kit (TOYO B-Net, Tokyo, Japan). Production of WT and mutant SOX11 proteins was assessed by immunoblot analysis with monoclonal anti-FLAG M2 HRP antibody (1:3,000; Sigma), following the manufacturer’s instructions. Morpholino and mRNA microinjection Antisense translation-blocking morpholinos (MOs) for sox11a —(5′-CGCTGTTGTCCGTTTGCTGCACCAT-3′), sox11b —(5′-CTGTGCTCCGTCTGCTGCACCATGT-3′) [17] , tp53 —(5′-GCGCCATTGCTTTGCAAGAATTG-3′) [18] and standard control—(5′-CCTCTTACCTCAGTTACAATTTATA-3′) MO were obtained from GeneTools (Philomath, OR) and injected (or co-injected) into one- to two-cell-stage embryos at a final concentration of 0.1 or 0.2 mM. In rescue assays, capped human SOX11 mRNAs transcribed in vitro from pEF6/V5-His B constructs were prepared using the mMessage mMachine T7 ULTRA Transcription Kit (Ambion, Carlsbad, CA), following the manufacturer’s instructions, and injected into one-cell-stage embryos. For each MO knockdown and rescue experiment, embryos from the same clutch were used as experimental subjects and controls. Approximately 1 μg of capped RNA was injected per embryo. The experiment was authorized by the institutional committee of fish experiments in the National Research Institute of Fisheries Science. Cell death detection To detect apoptotic cells in live embryos, embryos at 30 hpf were manually dechorionated and incubated in acridine orange (2 μg ml −1 in egg water) at 28 °C for 1 h. After washing with egg water six times for 10 min each, embryos were anaesthetized with tricaine, mounted in 2% methylcellulose and examined by confocal microscopy. Apoptotic cells were also examined by the TUNEL assay, as previously described [26] . Embryos at 30 hpf, were fixed overnight in 4% PFA with PBS at 4 °C and stored in 100% methanol at −20 °C. Samples were incubated in 100% acetone at −20 °C for 20 min. Following fixation, the embryos were rinsed three times with PBS containing 0.1% Tween-20. Samples were then permeabilized by treatment with 0.5% Triton X-100 and 0.1% sodium citrate in PBS for 15 min. Embryos were subjected to the TUNEL assay by using the ApopTag Red in situ Apoptosis Detection Kit (Merck KGaA Millipore, Darmstadt, Germany) according to the manufacture’s instruction. Detection and quantitation of visible and fluorescent images All animals were photographed under the same conditions using a LSM510 confocal microscope (Carl Zeiss, Jena, Germany). In each animal, acridine orange-positive cells were quantitated using a selection tool in Adobe Photoshop, for a colour range chosen by green colour selection of regions showing visually positive acridine orange staining. For analysis of embryos, defined head regions were selected in each embryo. Following pixel selection, a fuzziness setting of 0 was used, and chosen pixel numbers calculated using the image histogram calculation. Whole-mount immunohistochemistry For HuC/D staining, embryos at 48 hpf were fixed in 4% PFA overnight at 4 °C and dehydrated in methanol at −20 °C. For acetylated tubulin staining, embryos at 48 hpf were fixed in Dent’s fixative (80% methanol and 20% dimethyl sulphoxide) overnight at 4 °C. Embryos were permeabilized with proteinase K followed by postfixation with 4% PFA and washed with PBSTX (PBS containing 0.5% Triton X-100). After treating with 4% normal goat serum (NGS) in PBSTX for 2 h at room temperature, embryos were incubated with mouse anti-HuC/D (1:500, A21271, Life Technologies Co.) or mouse anti-acetylated tubulin (1:1,000, T7451, Sigma) antibodies in 4% NGS/PBSTX overnight at 4 °C. Embryos were washed five times with PBSTX for 10 min each and incubated with goat anti-mouse fluorescein isothiocyanate secondary antibody diluted in 2% NGS/PBSTX for 2 h at room temperature. After washing five times for 10 min each, embryos were mounted in 2% methylcellulose and examined using a Fluoview FV1000-D confocal microscope (Olympus). Accession codes: Exome sequence data for CSS patients have been deposited in the Human Genetic Variation Browser under the accession code HGV0000001 ( http://www.genome.med.kyoto-u.ac.jp/SnpDB/repository/HGV0000001.html ). Access to this data is controlled by the Yokohama City University Data Access Committee. How to cite this article: Tsurusaki, Y. et al. De novo SOX11 mutations cause Coffin–Siris syndrome. Nat. Commun. 5:4011 doi: 10.1038/ncomms5011 (2014).